Merging rhodium-catalysed C–H activation and hydroamination in a highly selective [4+2] imine/alkyne annulation Catalytic C–H activation and hydroamination represent two important strategies for eco-friendly chemical synthesis with high atom efficiency and reduced waste production. Combining both C–H activation and hydroamination in a cascade process, preferably with a single catalyst, would allow rapid access to valuable nitrogen-containing molecules from readily available building blocks. Here we report a single metal catalyst-based approach for N-heterocycle construction by tandem C–H functionalization and alkene hydroamination. A simple catalyst system of cationic rhodium(I) precursor and phosphine ligand promotes redox-neutral [4+2] annulation between N–H aromatic ketimines and internal alkynes to form multi-substituted 3,4-dihydroisoquinolines (DHIQs) in high chemoselectivity over competing annulation processes, exclusive cis -diastereoselectivity, and distinct regioselectivity for alkyne addition. This study demonstrates the potential of tandem C–H activation and alkene hydrofunctionalization as a general strategy for modular and atom-efficient assembly of six-membered heterocycles with multiple chirality centres. In recent years, transition metal-mediated C–H bond activation has been increasingly explored in catalytic construction of heterocycles that involve tandem formation of carbon–carbon and carbon–heteroatom bonds [1] , [2] , [3] , [4] , [5] , [6] , [7] , [8] . A major strategy for such catalytic heterocycles synthesis via C–H activation is the intermolecular coupling between aromatic compounds and alkynes to form six-membered benzoheterocycles ( Fig. 1a ). These [4+2] annulations utilize a variety of heteroatom-based ortho -directing groups for aromatic C–H bond activation. The resulting metallacycle intermediates ( A ) undergo subsequent alkyne coupling and ring-closure steps to incorporate the directing groups into the heterocyclic product backbone [9] , [10] , [11] . A dominant majority of these domino processes occur in the form of oxidative annulation that retains a carbon–carbon double bond in the heterocycle structure ( Fig. 1b ) [8] , [12] , [13] , [14] , [15] , [16] , [17] , [18] , [19] , [20] , [21] , [22] , [23] , [24] , [25] , [26] , [27] , [28] , [29] , [30] , [31] , [32] , [33] , [34] . For heteroatom-based directing groups with a N–H or O–H moiety, stoichiometric amounts of Ag(I) or Cu(II) oxidants are commonly used for oxidative [4+2] annulations. This need for external oxidants can be eliminated either by developing aerobic oxidation [25] , [26] , [27] , [34] or dehydrogenative coupling conditions [30] , or by using an ‘oxidizing directing group’ as the internal oxidant that releases a small molecule byproduct such as water [17] , [21] , alcohol [18] or carboxylic acid [23] , [33] . In principle, redox-neutral [4+2] annulations with aromatic compounds and alkynes would provide direct access to partially saturated benzoheterocycles in 100% atom efficiency and forms up to two new chirality centres ( Fig. 1a ). However, this strategy was only demonstrated in a single report in 2013 by Sun, Wang and coworkers [35] , who developed a Re(I)–Mg(II) bimetallic catalyst for benzamide/alkyne coupling to synthesize 3,4-dihydroisoquinolinones with controlled cis - or trans -diastereoselectivity ( Fig. 1c ). This redox-neutral [4+2] annulation featured a ring-closure step of Mg-catalysed intramolecular alkene addition by the amide N–H bond, which represents an example of main group metal-catalysed alkene hydroamination [36] . 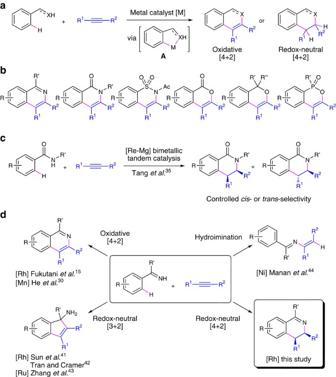Figure 1: Transition metal-catalyzed [4+2] annulations and related strategies. (a) Catalytic [4+2] annulations between aromatic compounds and alkynes via cyclometalated intermediates (A); XH=H-substituted σ-donating functional group to direct aromatic C–H activation at theortho-position. (b) Reported benzoheterocycle products from oxidative [4+2] annulations with NH or OH directing groups. (c) A Re–Mg bimetallic catalyst system for redox-neutral [4+2] annulation between benzamides and alkynes. (d) Divergent catalytic couplings between N–H aromatic ketimines and alkynes. Figure 1: Transition metal-catalyzed [4+2] annulations and related strategies. ( a ) Catalytic [4+2] annulations between aromatic compounds and alkynes via cyclometalated intermediates ( A ); XH=H-substituted σ-donating functional group to direct aromatic C–H activation at the ortho -position. ( b ) Reported benzoheterocycle products from oxidative [4+2] annulations with NH or OH directing groups. ( c ) A Re–Mg bimetallic catalyst system for redox-neutral [4+2] annulation between benzamides and alkynes. ( d ) Divergent catalytic couplings between N–H aromatic ketimines and alkynes. Full size image Considering that late transition metal catalysts have been widely used in both C–H activation and alkene hydroamination processes [1] , [36] , [37] , we envisioned that redox-neutral [4+2] annulations for N-heterocycle synthesis may be promoted by a single transition metal catalyst via a domino sequence of C–H bond activation, C–C bond formation by alkyne coupling and C–N bond formation by intramolecular alkene hydroamination. This ‘one catalyst does it all’ approach for redox-neutral annulations would complement existing methods with operationally simple procedures and provide opportunities for ligand-enabled control over chemo- and stereoselectivity for hydroamination. From the reaction mechanism perspective, our strategy can be compared with ruthenium- and gold-catalysed synthesis of 1,2-dihydroquinoline derivatives by 3-component coupling between an aromatic amine and two alkynes [38] , [39] , [40] . This redox-neutral [3+2+1] annulation involves a tandem sequence of intermolecular alkyne hydroamination and aromatic C–H functionalization. In the current study, we have focused our attention on metal-catalysed intermolecular couplings between N–H aromatic ketimines and internal alkynes ( Fig. 1d ). We and others have previously reported three classes of couplings between these two reaction partners to selectively form isoquinolines by oxidative [4+2] N-heterocyclization [15] , [30] , indene-based tertiary carbinamines by [3+2] carbocyclization [41] , [42] , [43] , and 2-aza-1,3-butadienes by alkyne hydroamination with N–H imine nucleophile (hydroimination) [44] . These divergent catalytic processes attest to the challenge of targeting desired redox-neutral [4+2] annulation with high chemoselectivity. We herein describe a mechanism-based development of a rhodium-catalysed redox-neutral [4+2] annulation with aromatic N–H ketimines and internal alkynes to form 3,4-dihydroisoquinolines (DHIQs), which are synthetic intermediates towards valuable 1,2,3,4-tetrahydroisoquinoline (THIQ) structures [45] . The strategic combination of a cationic Rh(I) catalyst precursor and a bis(phosphine) ligand enables this N-heterocyclization to proceed with high chemoselectivity over other possible coupling processes and exclusive diastereoselectivity for cis -3,4-disubstituted products. Regio- and stereochemistry results, as well as results from deuterium-labelling studies, are most consistent with a domino sequence of imine-directed aromatic C–H bond activation via oxidative addition, alkyne coupling, and a novel intramolecular alkene hydroimination. Synthetic utility of target DHIQ products are demonstrated with several stoichiometric and catalytic transformations including diastereoselective hydride reduction and Rh(III)-mediated regioselective C–H functionalizations. Initial observations and mechanistic implications Our study began with the detection of three annulation products from catalytic coupling between N–H aromatic ketimines and internal alkynes (Scheme 2a). In particular, Rh(I)-catalysed 1:1 coupling between benzophenone imine ( 1a ) and diphenylacetylene ( 2a ) led to formation of [3+2] carbocyclization product 3a (refs 41 , 42 , 43 ), oxidative [4+2] N-heterocyclization product 4a (refs 15 , 30 ), and the desired dihydroisoquinoline product 5aa by redox-neutral [4+2] N-heterocyclization. The overall yield and chemoselectivity depended significantly on the choices of Rh(I) catalyst precursor, ancillary ligand and solvent for the reaction ( vide infra ). Thus, the major challenge for our catalyst development was to selectively promote formation of 5aa over byproducts 3a and 4a . In particular, we expected that formation of isoquinoline byproduct 4a would be highly competitive due to the strong thermodynamic driving force of aromatization. To this end, our effort was guided by an early observation that cationic Rh(I) precursors with non-coordinating counteranions, for example, [Rh(cod) 2 ]BF 4 ( 6 ), appeared to promote higher chemoselectivity for 5aa than neutral Rh(I) precursors with anionic ligands such as [Rh(cod) 2 (OH)] 2 . In addition, 5aa was detected exclusively as the cis -3,4-diphenyl diastereomer by 1 H NMR spectroscopy with a relatively small H(3)-H(4) coupling in 1 H NMR ( 3 J ∼ 6.0 Hz), which supported gauche cis - H(3)-H(4) and gauche cis -3,4-disubstitution relationships [30] , [43] , [46] . Combined with proposed reaction pathways for mechanistically relevant annulation processes [8] , [15] , [30] , [35] , [41] , [42] , [43] , these results led us to suggest an imine-directed C–H oxidative addition on cationic Rh(I) [47] , [48] , [49] to form a cyclometalated Rh(III) hydride A1 ( Fig. 2b , Path 1; see Supplementary Fig. 88 for a more detailed discussion) [9] . Alkyne insertion into the Rh–H linkage and subsequent C–C reductive elimination gave an alkyne hydroarylation product C , which we envisioned as a key intermediate for [4+2] annulation products ( vide infra ) [47] , [48] , [49] . Alternatively, a neutral Rh(I) catalyst precursor may promote a deprotonation-type C–H activation pathway, leading to a cyclometalated Rh(I) complex A2 (Path 2). Subsequent alkyne insertion into the Rh–C bond gave an imine-chelated Rh(I) alkenyl complex D (refs 10 , 11 ), which could lead to [3+2] carbocyclization product 3 by sequential intramolecular imine insertion into the Rh-alkenyl linkage and protonation of the resulting Rh(I) alkyl complex [41] , [42] , [43] . 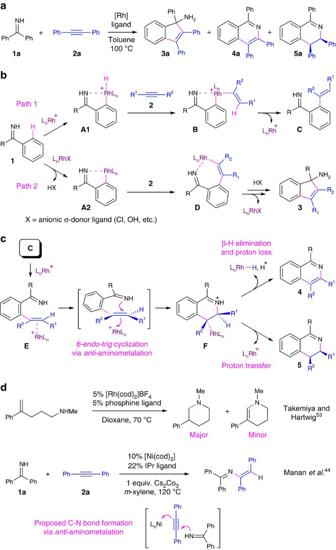Figure 2: Catalyst design for redox-neutral [4+2] imine/alkyne coupling. (a) Observation of three different annulation products with Rh(I) catalysts. (b) Proposed pathways for imine-directed aromatic C–H bond activation and subsequent alkyne coupling. (c) Proposed N-heterocyclization by intramolecular alkene hydroimination and subsequent competition between oxidative and redox-neutral [4+2] annulation product formations. (d) Mechanistically related reports on intramolecular alkene hydroamination and intermolecular alkyne hydroimination. Figure 2: Catalyst design for redox-neutral [4+2] imine/alkyne coupling. ( a ) Observation of three different annulation products with Rh(I) catalysts. ( b ) Proposed pathways for imine-directed aromatic C–H bond activation and subsequent alkyne coupling. ( c ) Proposed N-heterocyclization by intramolecular alkene hydroimination and subsequent competition between oxidative and redox-neutral [4+2] annulation product formations. ( d ) Mechanistically related reports on intramolecular alkene hydroamination and intermolecular alkyne hydroimination. Full size image Mechanism-based catalyst design The proposed acyclic intermediate C was not directly detected during our study. However, the involvement of similar alkyne hydroarylation intermediates was confirmed by Sun and Wang [35] in their recent report on Re(I)–Mg(II) bimetallic catalyst for redox-neutral [4+2] benzamide/alkyne annulation. In addition, Bergman, Ellman and coworkers have reported structurally analogous acyclic C–H alkenylation products in their reports on Rh(I)-catalysed N-heterocyclization with α,β-unsaturated N-benzyl imines and alkynes, which undergoes non-catalytic 6π-electrocyclization to form dihydropyridines as reactive intermediates for several one-pot procedures towards pyridine and tetrahydropyridine synthesis [49] , [50] , [51] . Aiming for a single catalyst-based domino procedure, we hypothesized that a cationic Rh(I) catalyst for the stage of C–H activation and alkyne coupling ( Fig. 2b , Path 1) could also promote subsequent ring closure by intramolecular alkene hydroamination. As described in Fig. 2c , alkene π-complexation between C and a Lewis acidic Rh(I) centre would promote intramolecular nucleophilic attack by the N–H imine moiety in stereospecific 6-endo-trig fashion to give metal alkyl intermediate F . With the stereochemistry of C–N bond formation determined by such anti -aminometalation [36] , [37] , F could undergo either syn -β-H elimination to give isoquinoline 4 or protonation of the Rh-alkyl linkage with stereospecific retention to give the cis -isomer of redox-neutral annulation product 5 (see Supplementary Fig. 88 for a more detailed description). Thus, we envisioned that an ideal catalyst system for selective synthesis of DHIQs should effectively promote a tandem sequence of C–H alkenylation ( 1 → C ), intramolecular alkene hydroamination ( C → F ), and selective protonation of a Rh-alkyl complex ( F → 5 ) over β-H elimination. This catalysis design is inspired by cationic Rh(I) catalysts that have been successfully explored by the Hartwig group for inter- and intramolecular alkene hydroamination [52] , [53] , [54] , [55] . For example, [Rh(cod) 2 ]BF 4 ( 6 ) was demonstrated as an effective catalyst precursor for anti -Markovnikov intramolecular hydroamination of vinylarenes with secondary aliphatic amines ( Fig. 2d ) [53] . Notably, selective formation of desired hydroamination products versus oxidative amination products in this report was significantly affected by the choice of chelating bis-phosphine ligands. Such ligand-controlled chemoselectivity can be attributed to the ligand bite angle effects on β-H elimination versus protonation of metal alkyl intermediates in several catalytic processes including alkene hydroamination versus oxidative amination, as well as Heck–Mizoroki olefinations versus the corresponding alkylation processes [56] . It is also noteworthy that we have recently reported a nickel-catalysed intermolecular alkyne hydroamination with N–H aromatic ketimines that proceeded by a proposed imine nulcleophilic attack on Ni(0)-coordinated alkyne for stereospecific anti -addition [44] . This result serves as an indirect evidence to support both the unconventional role of N–H imine moiety as a N-nucleophile for hydroamination and the proposed stereochemistry for C–N bond formation in current study. Catalyst development With mechanistic insights described above, we have focused our attention on the combination of cationic Rh(I) precursors and chelating bis-phosphine ligands for catalyst development ( Table 1 ). A particularly effective catalyst system was discovered using [Rh(cod) 2 ]BF 4 precursor ( 6 ) and DPEphos ligand (bis[(2-diphenylphosphino)phenyl] ether, 7 ). It is noteworthy that DPEphos is a prominent example of bis-phosphine ligands with wide bite angles, whose significant ligand effects on chemo- and regioselectivity in metal-catalysed coupling reactions including hydroamination are well documented [52] , [56] . At 100 °C and in toluene solvent, a 1:1 coupling between 1a and 2a was promoted by 5 mol% [Rh(cod) 2 ]BF 4 ( 6 ) and 6 mol% DPEphos ( 7 ) to selectively form 5aa in 93% yield over 24 h. Under these conditions, oxidative [4+2] annulation product 4a was formed in 3% yield, and the [3+2] carbocyclization product 3a was not detected (entry 1). Significantly reduced reactivity and chemoselectivity was observed when replacing DPEphos with various bis- and mono-phosphines (entries 2–8), or replacing 6 with several other Rh(I) catalyst precursors (entries 9–12). Switching from toluene to THF solvent led to similar overall reactivity but slightly lower selectivity for 5aa (entry 13), while much lower reactivity and chemoselectivity was observed in hexane (entry 14) and several solvents of higher polarity (entries 15–17). Lastly, using an increased amount of DPEphos ligand (entry 18) or reduced catalyst loading (entry 19) both led to lower combined yield of 5aa and 4a but higher yield for 4a formation. This observation suggested that the oxidative [4+2] annulation may also proceed in different pathways that involve non-catalytic ring-closure steps such as 6π-electrocyclization (see Supplementary Fig. 88 for a more detailed discussion on possible pathways for imine/alkyne coupling). Table 1 Optimization of conditions for redox-neutral [4+2] imine/alkyne annulation. Full size table Alkyne substrate scope With the standard reaction conditions established, various aromatic N–H ketimine ( 1 ) and internal alkyne ( 2 ) substrates were studied for Rh(I)-catalysed redox-neutral [4+2] annulation (Scheme 3). In general, 1,3,4-trisubstiuted DHIQs ( 5 ) were formed in exclusive cis -3,4-diastereoselectivity and high chemoselectivity, with only trace amounts (0–5%) of isoquinoline byproducts ( 4 ) and no detection of indenamine byproducts ( 3 ) as evidenced by gas chromatography (GC) and 1 H NMR analysis of the unpurified reaction mixture. However, several DHIQ products appeared to undergo spontaneous dehydrogenation during the separation and purification procedures, which generated small amounts of isoquinoline byproducts 4 that could not be fully removed from the isolated DHIQ products 5 ( vide infra ). Scope of the alkyne substrates was studied with benzophenone imine ( 1a ) as the reaction partner, and high coupling yields were achieved with various symmetrical alkynes having aryl, 2-thienyl, and alkyl substituents (products 5aa – 5am ). However, no coupling products were detected for bis(2-pyridyl)acetylene or terminal alkynes such as phenylacetylene. Reactions with non-symmetrical phenyl alkyl alkynes led to the exclusive formation of cis -3-alkyl-4-phenyl products ( 5an – 5ap ). By sharp contrast, most reported methods of oxidative [4+2] heterocyclization with non-symmetrical aryl alkyl akynes displayed the opposite regioselectivity [8] , [12] , [13] , [14] , [15] , [16] , [17] , [18] , [19] , [20] , [21] , [22] , [23] , [24] , [25] , [26] , [27] , [28] , [29] , [30] , [31] , [32] , [33] , [34] . For instance, regioselective formation of a 3-aryl-4-alkyl-substituted isoquinoline product was recently reported by the Wang group by manganese-catalysed dehydrogenative [4+2] annulation of N–H imines and alkynes [30] . The only example of similar regioselectivity with aryl alkyl alkynes was reported by the Cramer group on rhodium(III)-catalysed oxidative [4+2] annulation of N-acyl arylsulfonamides and alkynes, which promoted formation of a 3-alkyl-4-aryl-substituted benzosultam product in modest regioselectivity (2:1) (ref. 27 ). The reaction with 1-(2-thienyl)-2-phenylacetylene generated a 4:1 mixture of regioisomers, and the major isomer of 3-phenyl-4-(2-thienyl)-substituted DHIQ product 5aq was isolated in 66% yield. This modest regioselectivity was likely affected by potential coordination between sulfur centre of the 2-thienyl moiety and the cationic Rh(I) centre during the akyne coupling process. Due to product decomposition by dehydrogenation, isolated products 5am – 5ao were contaminated with ∼ 10–15% of the corresponding isoquinoline byproducts, and the reported yields were estimated by 1 H NMR analysis (see Supplementary Figs 29, 31 and 33 for more details). N–H ketimine substrate scope Scope of the ketimine substrates was studied by coupling with diphenylacetylene ( 2a ), and high reactivity was observed for both diaryl and aryl alkyl ketimines with phenyl groups ( 5ia and 5ja ) or electron-poor aryl groups having F, Cl and CF 3 groups at para or meta positions ( 5ba , 5ca , 5fa and 5ka – 5oa ). Electron-rich di( p -tolyl) N–H ketimine gave product 5da in 70% yield, while di( p -anisyl) N–H ketimine failed to react with 2a to give detectable coupling products. Such electronic effect on ketimine reactivity was further demonstrated with product 5ga , which was formed with exclusive regioselectivity for C–H functionalization of the electron-poor aryl group with meta -CF 3 substituent over the electron-rich one with meta -methoxy substituent. Notably, the sterically hindered di( o -tolyl) N–H ketimine did react with 2a to give redox-neutral [4+2] adduct 5ha . Product decomposition via dehydrogenation was also observed for 5ha , and an isolated yield of 66% was calculated based on 1 H NMR analysis (see Supplementary Fig. 54 for details). The solid-state structures of products 5aa , 5an and 5na were established by single-crystal X-ray diffraction analysis, which confirmed the cis -diastereoselectivity and 3-alkyl-4-aryl regioselectivity for corresponding DHIQ products. Current results of the substituent effects on coupling reactivity and regioselectivity provide several mechanistic insights that were consistent with the proposed pathway for C–H alkenylation ( Fig. 2b , Path 1). Firstly, the lack of significant reactivity dependence on symmetrically substituted alkyne substrates (products 5aa – 5am ) suggested that the proposed C–C and C–N bond formation steps ( B → C , E → F ) were not rate determining. Secondly, the highly regioselective functionalization at the more electron-deficient aryl moiety in product 5ga suggested a C–H activation pathway that does not involve electrophilic aromatic substitution [1] . Instead, these restuls were consistent with a proposed rate-determining step of C–H oxidative onto the Rh(I) centre of the catalyst ( 1 → A1 ) (ref. 49 ). Thirdly, the distinct regioselectivity with non-symmetrical phenyl alkyl alkynes (products 5an – 5ap ) was consistent with proposed alkyne insertion into a Rh–H linkage, which placed the Rh centre preferentially at the more stabilized, α-to-phenyl position in intermediate B (R 1 =alkyl, R 2 =phenyl). Subsequent C–C reductive elimination gave Murai-type hydroarylation product C (refs 47 , 48 , 49 ), whose regiochemistry was reflected in the 3-alkyl-4-phenyl substitution pattern of the corresponding DHIQ product 5 . To further investigate regiochemistry of the proposed C–H alkenylation intermediate C , the current catalyst system was explored for a 1:1 coupling between 2-phenylpyridine and n -butylphenylacetylene that should not give an annulation product without oxidants ( Fig. 4a ) [10] , [57] . Under the standard conditions for catalytic redox-neutral [4+2] annulations, a ( E )-1,1-diarylhexene product 8 was acquired in 83% yield and with exclusive regio- and stereoselectivity (see Supplementary Figs 75 and 77 for 1H NMR and NOESY spectra). This result is consistent with our proposed C–H alkenylation pathway and represents a relatively rare example of high selectivity towards 1,1-diarylalkene regioisomers for catalytic hydroarylation with aryl alkyl alkynes by the directed C–H activation strategy [21] , [58] . Lastly, the failure of produt formation for the highly electron-rich imine substrate di(p-anisyl) N–H ketimine (product 5ea ) suggested that C–H activation may be inhibited by strong σ-complexation between Rh(I) and imine ligands. A similar lack of reactivity for electron-rich N–H aromatic imines was observed in our previous study on Ni-catalysed hydroimination of alkynes [44] . 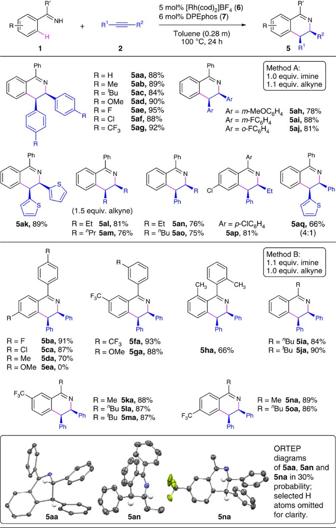Figure 3: Scope of Rh-catalyzed redox-neutral [4+2] imine/alkyne annulation. General reaction conditions:1(0.28 mmol for Method A, 0.31 mmol for Method B),2(0.31 mmol for Method A, 0.28 mmol for Method B); [Rh(cod)2]BF4(6, 5.0 mol%), DPEphos (7, 6.0 mol%), toluene (1.0 ml), 100 °C, 24 h; averaged yield of isolated products from two runs. Figure 3: Scope of Rh-catalyzed redox-neutral [4+2] imine/alkyne annulation. General reaction conditions: 1 (0.28 mmol for Method A, 0.31 mmol for Method B), 2 (0.31 mmol for Method A, 0.28 mmol for Method B); [Rh(cod) 2 ]BF 4 ( 6 , 5.0 mol%), DPEphos ( 7 , 6.0 mol%), toluene (1.0 ml), 100 °C, 24 h; averaged yield of isolated products from two runs. 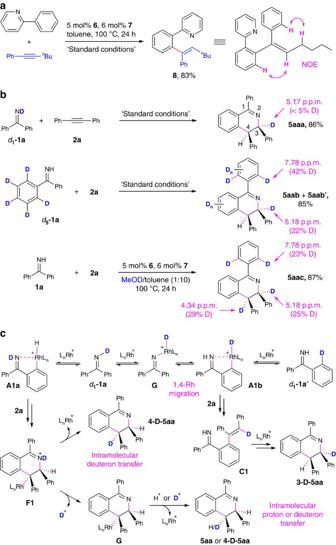Figure 4: Reaction mechanism studies and analysis. (a) Regioselective alkyne hydroarylation with 2-phenylpyridine under standard catalytic conditions for [4+2] imine/alkyne annulation. (b) Results from deuterium-labelling studies. (c) Proposed pathways for regioselective deuterium transfer and equilibrium processes for H/D scrambling. Full size image Figure 4: Reaction mechanism studies and analysis. ( a ) Regioselective alkyne hydroarylation with 2-phenylpyridine under standard catalytic conditions for [4+2] imine/alkyne annulation. ( b ) Results from deuterium-labelling studies. ( c ) Proposed pathways for regioselective deuterium transfer and equilibrium processes for H/D scrambling. Full size image To better understand hydrogen atom transfer processes in the proposed mechanism for redox-neutral [4+2] annulation ( Fig. 2b,c ), we carried out deuterium-labelling studies on the formation of 5aa by coupling between 1a and 2a under standard catalytic conditions and with various deuterium sources ( Fig. 4b ). Firstly, the reaction with Ph 2 C=ND ( d 1 -1a ) led to <5% D incorporation at C3 position of the product 5aaa . The significant deuterium loss suggested a rapid hydrogen/deuterium (H/D) srambling between the imine moiety and the reaction media, presumably due to traces of moisture or acid impurities. The regioselective D-transfer to C3, albeit in low conversion, suggested an intramolecular H/D exchange between the imine N centre and the ortho aromatic positions of d 1 -1a . The resulting ortho -D atom would migrate to C3 position of 5aa by the proposed pathways for C–H alkenylation ( Fig. 2b ) and intramolecular alkene hydroamination ( Fig. 2c ). Secondly, the reaction with (C 6 D 5 )PhC=NH ( d 5 -1a ) led to an inseparable mixture of products 5aab and 5aab′ via imine-directed C–H or C–D activation. This mixture displayed 22% D incorporation at C3 position, while 42% D could be measured at each ortho -position of the 1-phenyl group. This result further supported the proposed H/D exchange between the N centre and ortho aromatic positions of imine substrates. Thirdly, the reaction with non-deuterated 1a and in a mixed solvent of 1:10 MeOD/toluene gave 5aac with 25% D at C3, 29% D at C4 and 23% D at each ortho -position of the 1-phenyl group. The partial deuterium incorporation at C4 suggested that the cleavage of Rh-alkyl linkage ( Fig. 2c , F → 5 ) likely occurred by both intra- and intermolecular proton/deuterium transfer processes. Despite the complication by facile H/D scrambling, results from these deuterium-labelling experiments allowed us to gain further evidence and additional details for proposed reaction pathways as described in Fig. 4c . The proposed H/D exchange between the imine N atom and ortho aromatic positions likely occurs by reversible N–H(D) oxidative addition onto Rh(I) centre of the catalyst to form a Rh(III) hydrido iminyl intermediate ( d 1 -1a → G ), which undergoes reversible 1,4-Rh migration [59] to activate an ortho aromatic C–H bond and form the cyclometalated intermediate A1b with a Rh–D linkage. Subsequent C–D reductive elimination generates ortho -deuterated imine ( d 1 -1a′ ) and completes the proposed H/D exchange. Notably, the cyclometalated Rh(III) intermediate with a Rh–D linkage that is analogous to A1b is also formed by imine-directed ortho C–D activation (that is, microscopic reverse of C–D reductive elimination) with d 5 -1a ( Fig. 2b ). As described in Path 1 in Fig. 2b , a tandem sequence of alkyne insertion with A1b (or its analogue from d 5 -1a ) and C–C reductive elimination leads to regioselective D-transfer onto the mono-substituted alkenyl position in alkyne hydroarylation product C1 , which followed the proposed hydroamination pathway ( Fig. 2c , C → 5 ) to form the 3-deuterated compound 3-D-5aa as observed in products 5aaa – 5aac . Besides the proposed intramolecular H/D exchange ( d 1 -1a → d 1 -1a′ ), imine-directed ortho C–H oxidative addition forms the cyclometalated intermediate A1a that transforms into intermediate F1 after the proposed alkyne coupling and ring-closure steps. With the D atom retained on the iminium N centre in F1 , cleavage of the Rh-alkyl linkage by intramolecular deuteron transfer in stereospecific retention forms the 4-deuterated compound 4-D-5aa as observed in product 5aac . Alternatively, deuteron dissociation from F1 and subsequent cleavage of the Rh-alkyl linkage by intermolecular proton or deuteron transfer forms the non-deuterated 5aa or 4-D-5aa respectively. The observed facile H/D scrambling can be attributed to the Bronsted acid behaviours by several proposed reactive intermediates such as cationic Rh(III) hydride/deuteride complexes ( A1a , A1b and G ) and the iminium species ( F1 and its protonated analogue), which could undergo fast and reversible H/D transfer with external proton or deuteron sources such as trace moisture, acid, or added MeOD in the reaction environment. Product 5aa was subjected to several stoichiometric and catalytic transformations to explore DHIQ products from the current study as valuable building blocks in chemical synthesis ( Fig. 5 ). In particular, we expected that hydrogenation or nucleophilic addition of the imine moiety in these DHIQ products could lead to stereoselective formation of the corresponding THIQs, which are important structural motifs in biologically active compounds including natural alkaloids and drug molecules [45] . Thus, we studied the hydride reduction of 5aa using a procedure reported by Bergman and Ellman ( Fig. 5a ) [51] . Upon acid-mediated activation, 5aa underwent a borohydride reduction to give a 20:1 mixture of two diastereomers of the corresponding THIQ product in 87% overall yield. 1 H NMR and X-ray crystallography indicated that the major product was the all- cis -diastereomer ( 9a ), while the minor stereoisomer 9b displayed cis -1,3 and trans -3,4 stereochemistry. The cis -1,3 relationship in both isomers should result from stereospecific, anti to 3-phenyl hydride transfer [51] . The formation of 9b was likely due to acid-mediated epimerization at C3 via iminium intermediates [60] , [61] . This result highlights the pontential of redox-neutral [4+2] imine/alkyne annulation as a new approach towards stereoselective synthesis of poly-substituted THIQs that complements existing strategies such as intramolecular electrophilic aromatic substitutions [62] or metal-catalysed enantioselective hydrogenation of isoquinolines [63] , [64] . 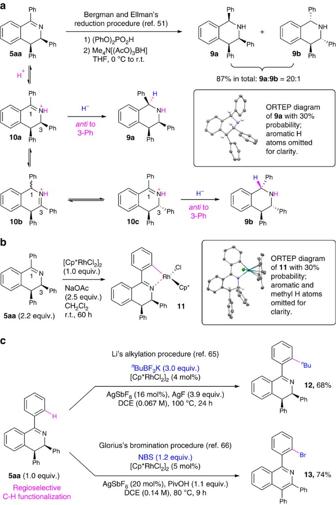Figure 5: Demonstration of synthetic transformations of DHIQ products with the model compound 5aa. (a) Diastereoselective hydride reduction. (b) Rh(III)-mediated regioselective cyclometalation. (c) Rh(III)-catalyzed aromatic functionalizations via directed C–H activation. Figure 5: Demonstration of synthetic transformations of DHIQ products with the model compound 5aa. ( a ) Diastereoselective hydride reduction. ( b ) Rh(III)-mediated regioselective cyclometalation. ( c ) Rh(III)-catalyzed aromatic functionalizations via directed C–H activation. Full size image To explore 1-aryl-substituted DHIQs as aromatic imine analogues for imine-directed C–H functionalization, a 1:1 reaction between 5aa and a Cp*-ligated Rh(III) complex [Cp*RhCl 2 ] 2 was carried out at room temperature with sodium acetate as an additive ( Fig. 5b ). Although this transformation occurred with incomplete conversion, we were able to isolate a Rh(III) product with a cyclometalated DHIQ ligand ( 11 ) and characterized its solid-state structure by single-crystal X-ray diffraction. This {Cp*RhCl[η 2 -(C,N)-DHIQ]} complex resulted from regioselective C–H activation of 5aa at the ortho -position of 1-phenyl instead of 3-phenyl substituent. Notably, a preliminary test reaction between the oxidative [4+2] annulation product 4a and [Cp*RhCl 2 ] 2 under similar conditions failed to generate cyclometalation products. Such reactivity difference between 5aa and 4a may result from the more rigid structure of isoquinoline than DHIQ, which led to more significant steric crowding by phenyl substituents and 1- and 3-positions that inhibits imine-directed aromatic C–H activation. The Rh(III)-mediated regioselective C–H activation with 5aa was further exploited in two catalytic transformations following reported procedures by Li [65] and Glorius [66] , both using [Cp*RhCl 2 ] 2 as the catalyst precursor ( Fig. 5c ). A coupling between 5aa and the organoboron reagent n BuBF 3 K gave alkylated DHIQ product 12 in 68% yield [65] . Consistent with the stoichiometric cyclometalation result ( Fig. 5b ), the n -butyl group was attached selectively at an ortho -position of the 1-phenyl group. Notably, the cis -3,4-diphenyl stereochemistry of the DHIQ backbone was retained in both compounds 11 and 12 . By contrast, 5aa underwent C–H bromination with the NBS reagent in same regioselectivity but dehydrogenated under the reaction conditions to give brominated isoquinoline product 13 in 74% yield [66] . Although it is difficult to rationalize the observation of such dehydrogenation under non-oxidation conditions without a systematic investigation, this result resonates with the recent report by the Wang group on Mn-catalysed dehydrogenative [4+2] imine/alkyne annulation for isoquinoline synthesis [30] . In another preliminary reactivity evaluation, we found that the isoquinoline compound 4a failed to undergo C–H bromination under similar reaction conditions to form 13 , presumably due to the steric hindrance against cyclometalation as previously discussed. Thus, DHIQ products from current study could also be explored as isoquinoline precursors by tandem functionalization-dehydrogenation strategy. In summary, we have developed a single catalyst-based approach towards atom-efficient N-heterocycle construction by tandem C–H activation, alkyne coupling, and intramolecular alkene hydroamination. The mechanism-based catalyst development led to the combination of a cationic Rh(I) catalyst precursor and a bis(phosphine) ligand DPEphos, which promotes a redox-neutral [4+2] annulation between N–H aromatic ketimines and internal alkynes to form cis -3,4-disubstituted 3,4-dihydroisoquinolines (DHIQs) in high chemo-, regio- and stereoselectivity. With a proposed ligand-enabled intramolecular alkene hydroamination to introduce C3- and C4-chirality, this method can be potentially developed into an enantioselective version for asymmetric synthesis of poly-substituted chiral DHIQ building blocks towards highly valuable THIQ structures. The current strategy of combining metal-catalysed C–H functionalization and alkene hydrofunctionalization represents a unified synthetic approach towards various 6-membered benzoheterocycles by redox-neutral [4+2] annulation between aromatic compounds and alkynes. General procedure for redox-neutral [4+2] imine/alkyne annulations Into a 4 ml scintillation vial equipped with a magnetic stir bar was placed [Rh(cod) 2 ]BF 4 ( 6 , 5.6 mg, 0.014 mmol, 0.050 equiv. ), DPEphos ( 7 , 8.9 mg, 0.017 mmol, 0.060 equiv. ), and 1.0 ml of toluene. Next, N–H ketimine 1 (0.28 mmol, 1.0 equiv.) and internal alkyne 2 (0.31 mmol, 1.1 equiv.) were added into the vial for the synthesis of products 5aa – 5aq (demonstration of alkyne substrate scope). For the synthesis of products 5ba – 5oa (demonstration of imine substrate scope), 0.28 mmol alkyne 2 (1.0 equiv.) and 0.31 mmol of imine 1 (1.1 equiv.) were added instead. The vial was sealed with a silicone-lined screw-cap, transferred out of the glovebox, and stirred at 100 °C for 24 h. After the reaction mixture was cooled to room temperature, all volatile materials were removed under reduced pressure. Further purification was achieved by flash-column chromatography using neutral alumina. Yields of the isolated products are based on the average of two runs under identical conditions. The exclusive cis -diastereoselectivity for products was determined by GC and 1 H NMR analysis of the unpurified reaction mixture. See Supplementary Figs 1–87 and Supplementary Methods for full experimental details and analytical data for characterization of new compounds. Accession codes: The X-ray crystallographic coordinates for structures reported in this study have been deposited at the Cambridge Crystallographic Data Centre (CCDC), under deposition numbers 1424375-1424378 (compounds 5aa , 9a , 5na and 11 ) and 1442483 (compound 5an ). These data can be obtained free of charge from The Cambridge Crystallographic Data Centre via www.ccdc.cam.ac.uk/data_request/cif . How to cite this article: Manan, R. S. et al. Merging rhodium-catalysed C–H activation and hydroamination in a highly selective [4+2] imine/alkyne annulation. Nat. Commun. 7:11506 doi: 10.1038/ncomms11506 (2016).